Circadian rhythms of hydraulic conductance and growth are enhanced by drought and improve plant performance Circadian rhythms enable plants to anticipate daily environmental variations, resulting in growth oscillations under continuous light. Because plants daily transpire up to 200% of their water content, their water status oscillates from favourable during the night to unfavourable during the day. We show that rhythmic leaf growth under continuous light is observed in plants that experience large alternations of water status during an entrainment period, but is considerably buffered otherwise. Measurements and computer simulations show that this is due to oscillations of plant hydraulic conductance and plasma membrane aquaporin messenger RNA abundance in roots during continuous light. A simulation model suggests that circadian oscillations of root hydraulic conductance contribute to acclimation to water stress by increasing root water uptake, thereby favouring growth and photosynthesis. They have a negative effect in favourable hydraulic conditions. Climate-driven control of root hydraulic conductance therefore improves plant performances in both stressed and non-stressed conditions. The circadian rhythm causes the oscillation of the transcript abundance of 5–15% of plant genes [1] , [2] , [3] , [4] and the rhythmic variations of leaf expansion rate under continuous light (rhythmic growth) [5] , [6] , [7] . This rhythm, entrained by environmental cues such as light and temperature [4] , [8] , provides a competitive advantage to plants able to anticipate daily environmental variations and to synchronize growth with them [4] , [8] , [9] , although the mechanisms for such improved plant performance are not known. The core oscillator, well-described in Arabidopsis thaliana , is conserved in higher plants [10] and coordinates physiological mechanisms related to metabolism, growth and development [9] , [11] , [12] . In A. thaliana and other dicotyledons, oscillations of growth and gene expression are observed in continuous light with a period of about 24 h (refs 5 , 7 ). Paradoxically, cereals display circadian oscillations of gene expression [2] , [10] , but no rhythmic growth has so far been detected [6] , [13] . Plants transpire every day up to 200% of their water content (versus 1–2% for animals), so their water status oscillates from favourable during the night to unfavourable during the day, with amplitudes that increase with light, air vapour pressure deficit (VPD) and soil water deficit [14] . Leaf elongation rate (LER, largely independent of photosynthesis [14] ) essentially follows the same time course. In maize, large variations of LER are observed upon changes in soil water status or evaporative demand, with time constants of 30 min (ref. 15 ). This involves rapid changes in stomatal conductance and plant hydraulic conductivity, in particular in the activity of Plasma membrane Intrinsic Protein (PIP) aquaporins [16] , [17] , [18] , [19] . These rapid movements are synchronous with changes in turgor pressure [18] , whose effects are modulated by cell-wall mechanical properties via expansins and other cell-wall enzymes [20] . Light per se has no clear role on leaf growth of monocotyledons in natural conditions [14] . Furthermore, the (basal) growth zone of monocot leaves does not receive direct light signals because it is enclosed by the sheaths of older leaves, so light itself might be insufficient to trigger rhythmic growth in these species [6] , [13] as it does in A. thaliana [5] , [7] . We have investigated whether day/night alternations of plant water status during an entrainment period (EP, previous days before continuous light) induce an endogenous rhythm of maize leaf growth, questioned to what extent the control of rhythmic growth is hydraulic and investigated the ecological implications for plant performance. Experiments were performed in a novel phenotyping platform, allowing analysis of leaf growth and transpiration of a large number of plants in naturally fluctuating environmental conditions. Indeed, the absence of circadian rhythmic growth observed previously in maize and rice [6] , [13] could be due to a low evaporative demand during EP in standard growth chambers. We show here that the amplitude of rhythmic growth in continuous light depends on the severity of temporary water stress during the EP. It involves oscillations of plant hydraulic conductance and of transcript abundances of PIP aquaporins. A model suggests that this stress-dependent control of plant hydraulic conductance contributes to drought tolerance by facilitating water uptake in stressed conditions, whereas it is turned off in favourable water conditions because it has a negative intrinsic effect on growth and photosynthesis. LER oscillations depended on the EP LER oscillated in continuous light with large variations of amplitude between experiments ( Fig. 1 ). Stomatal conductance, transpiration rate and net photosynthesis rate did not clearly oscillate ( Supplementary Fig. 1 ), unlike the case in A. thaliana [9] . The nearly stable net photosynthesis rate also suggests the absence of photodamage and inhibition of photosystem II during the continuous light period [21] . The period of LER oscillations was 24 h regardless of experimental conditions (non-significant differences). 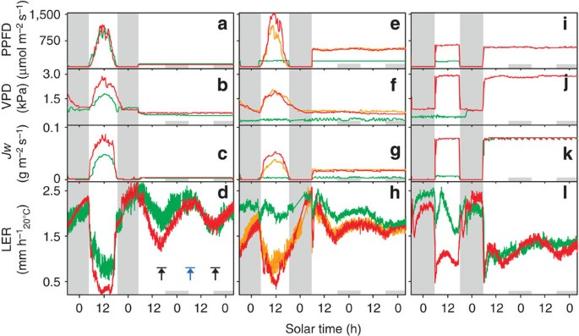Figure 1: The endogenous rhythm of leaf elongation rate in continuous light is linked to the entrainment period. (a,e,i) Photosynthetic photon flux density (PPFD). (b,f,j) Vapour pressure deficit (VPD). (c,g,k) Transpiration (Jw). (d,h,l) Leaf elongation rate (LER). (a–d) Entrainment period (EP) in green house at high (red) or low (green) evaporative demand (experiments 11 and 12). (e–h) EP either with low evaporative demand in a growth chamber (green, experiments 22) or high evaporative demand in green house (red and orange, experiments 9 and 8). (i–l) EP in growth chamber at high (red) or low (green) evaporative demands (experiments 20 and 21). Arrows indindicate the subjective dusks (black) and dawn (blue). Error bars either side of the solid line represent the confidence interval atP<0.05,n≥6 (Supplementary Table 1). The interval of time between subjective dusk and dawn (that is, times with minimum and maximum values of LER, respectively) varied from 11.5 to 15.5 h ( Supplementary Table 1 ) and was linearly related to the amplitude of LER variations during the EP ( Supplementary Fig. 2 ). Such a change in phase has been observed in A. thaliana as the result of the interplay between ABA signalling and the circadian clock [22] , [23] . Figure 1: The endogenous rhythm of leaf elongation rate in continuous light is linked to the entrainment period. ( a , e , i ) Photosynthetic photon flux density (PPFD). ( b , f , j ) Vapour pressure deficit (VPD). ( c , g , k ) Transpiration ( J w). ( d , h , l ) Leaf elongation rate (LER). ( a – d ) Entrainment period (EP) in green house at high (red) or low (green) evaporative demand (experiments 11 and 12). ( e – h ) EP either with low evaporative demand in a growth chamber (green, experiments 22) or high evaporative demand in green house (red and orange, experiments 9 and 8). ( i – l ) EP in growth chamber at high (red) or low (green) evaporative demands (experiments 20 and 21). Arrows in d indicate the subjective dusks (black) and dawn (blue). Error bars either side of the solid line represent the confidence interval at P <0.05, n ≥6 ( Supplementary Table 1 ). Full size image The amplitude of LER oscillations during continuous light was largest when plants were entrained with large oscillations of transpiration rate ( Fig. 1 ) and leaf water potential during EP ( Fig. 2 ). High evaporative demand during EP via increased air VPD caused high oscillation amplitudes during continuous light ( Fig. 1a–d ). High light intensity without change in VPD during EP caused smaller oscillation amplitudes of LER during continuous light, consistent with a smaller effect on transpiration and LER during EP. Maximum amplitudes of LER during continuous light were observed when both light and VPD had maximum amplitudes during EP ( Fig. 1e–h , red traces and Fig. 1i–l ). These tendencies applied to 21 experiments ( Supplementary Table 1 ), in which the amplitude during continuous light was closely related to that during EP ( Supplementary Fig. 3 ). A common relationship applied to all experiments with high evaporative demand during continuous light ( r =0.8), regardless of conditions during EP in either gradual (green house) or rapid (growth chamber) alternations of climatic conditions. It also applied to experiments in which the amplitude of LER oscillations during EP was manipulated via hydraulic conductivity in two different soils or in hydroponics ( Supplementary Fig. 3a ). This relationship was more tight when continuous light occurred with dry air (high VPD), thereby decreasing leaf water potential ( Supplementary Fig. 3a ), but was also observed with wetter air ( Supplementary Fig. 3b ). 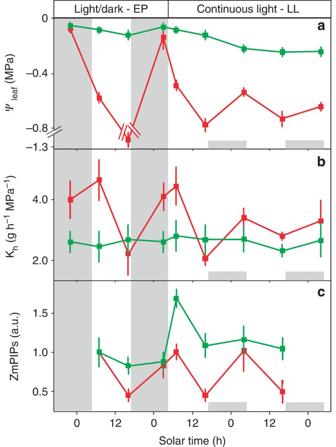Figure 2: The endogenous rhythm of leaf elongation rate is linked to variations in leaf water potential, plant hydraulic conductance and the expression level ofZmPIPaquaporins in roots. Experiments 9 and 22, LER presented inFig. 1, plants with either high (red) or low (green) evaporative demand during EP. (a) Leaf water potential. (b) Plant hydraulic conductance (Kh). (c) Mean expression of 12PIPs in roots. Values normalized by expression levels of eachZmPIPat 07:00 day 1. Error bars either side of the solid line represent the confidence interval atP<0.05,n=3 inc,n≥15 for other panels (Supplementary Table 1). Figure 2: The endogenous rhythm of leaf elongation rate is linked to variations in leaf water potential, plant hydraulic conductance and the expression level of ZmPIP aquaporins in roots. Experiments 9 and 22, LER presented in Fig. 1 , plants with either high (red) or low (green) evaporative demand during EP. ( a ) Leaf water potential. ( b ) Plant hydraulic conductance ( K h ). ( c ) Mean expression of 12 PIP s in roots. Values normalized by expression levels of each ZmPIP at 07:00 day 1. Error bars either side of the solid line represent the confidence interval at P <0.05, n =3 in c , n ≥15 for other panels ( Supplementary Table 1 ). Full size image Plants showing genetic differences in sensitivity to water deficit differed in oscillation amplitude of LER during continuous light ( Fig. 3 and Supplementary Fig. 4 ). This was the case for B73 plants introgressed with a genomic region that confers lower sensitivity to water deficit [24] , and to plants downexpressing the NCED/VP14 gene (AS) involved in ABA synthesis [19] . In both cases, oscillations of LER differed between lines during the EP (difference in sensitivity) and continuous light ( Fig. 3a,b ), suggesting a partly common mechanism of oscillations during EP and continuous light. 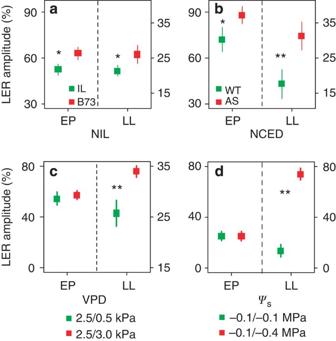Figure 3: The amplitude of LER oscillations increased with water stress and water flux through the plants. Compared amplitudes during the EP and continuous light for (a) plants introgressed with a genomic region that confers lower sensitivity to water deficit (experiment 2), (b) plants under-expressing theNCED/VP14gene (experiment 7), (c) plants with common environmental conditions during EP and grown with low (green) or high (red) evaporative demand during continuous light, (d) plants grown in hydroponics at −0.1 MPa during the EP, then at either −0.1 (green) or −0.4 MPa (red) during continuous light (experiment 18). Error bars either side of the solid line represent the confidence interval atP<0.05,n≥8 (Supplementary Table 1). *, ** represent significant difference,t-test atP-values <0.05 and 0.01. Figure 3: The amplitude of LER oscillations increased with water stress and water flux through the plants. Compared amplitudes during the EP and continuous light for ( a ) plants introgressed with a genomic region that confers lower sensitivity to water deficit (experiment 2), ( b ) plants under-expressing the NCED/VP14 gene (experiment 7), ( c ) plants with common environmental conditions during EP and grown with low (green) or high (red) evaporative demand during continuous light, ( d ) plants grown in hydroponics at −0.1 MPa during the EP, then at either −0.1 (green) or −0.4 MPa (red) during continuous light (experiment 18). Error bars either side of the solid line represent the confidence interval at P <0.05, n ≥8 ( Supplementary Table 1 ). *, ** represent significant difference, t -test at P -values <0.05 and 0.01. Full size image Core oscillator transcripts oscillated with no effect of EP We have performed a transcriptome analysis at night, subjective dusk and subjective dawn in the leaf growth zone of plants entrained with high daily alternations of leaf water potential, and compared it with the time course of transcript abundance in plants entrained in favourable conditions in this study or in a transcriptome analysis published earlier [2] . Among 38,534 tested putative genes, only 1% varied significantly during continuous light ( Supplementary Fig. 5 ). Transcript abundance of orthologue genes of the A. thaliana core oscillator [5] , [9] , [25] , [26] varied in continuous light, in particular GIGANTEA ( GI ) in both roots and leaves ( Fig. 4a–c ), with maximum and minimum values at subjective dusk and dawn, respectively. The transcript abundances of CIRCADIAN CYCLE ASSOCIATED1 ( CCA1 ), LATE ELONGATED HYPOCOTYL ( LHY ) and PSEUDO-RESPONSE REGULATORS ( PRR1 , PRR5 and PRR7) also showed alternations ( Fig. 4d–f ). Interestingly, the transcripts abundances of GI and CCA1 equally oscillated when plants were entrained with either high or low oscillations of transpiration during EP ( Fig. 4a–c,e ), suggesting that core oscillator genes did not directly respond to adverse hydraulic conditions during EP. The transcripts amount of an orthologue of the A. thaliana ABA-related gene ( ABAR/CHLH/GUN5 ) varied in opposite phase with PRR1 (also known as timing of the CAB expression 1 TOC1 (refs 27 , 28 , 29 ), as in A. thaliana [22] . This gene, proposed to favour water homoeostasis via a loop between TOC1 and ABA [22] , might play a role to coordinate plant hydraulic properties with the core oscillator. 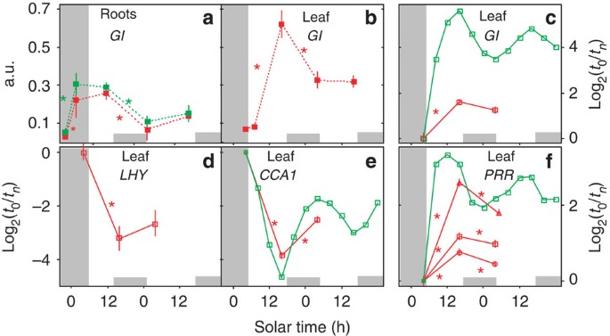Figure 4: Transcript abundance of core oscillator genes. Transcript abundance under high and low evaporative demands during EP (red and green lines, respectively). Solid lines represent microarray data (a,b), dotted lines represent qRT–PCR (c–f). (a)GIin roots (b)GIin leaves (c)GIin leaves (d)LHY(e)CCA1(f)PRRfamily genes. Circles representPRR1, triangles representPRR5, squares representPRR7. Data represented by green lines inc,e,fis from the study by Khanet al.2Error bars represent s.d.n=3. * represents significant difference in at-test,P<0.05. Figure 4: Transcript abundance of core oscillator genes. Transcript abundance under high and low evaporative demands during EP (red and green lines, respectively). Solid lines represent microarray data ( a , b ), dotted lines represent qRT–PCR ( c – f ). ( a ) GI in roots ( b ) GI in leaves ( c ) GI in leaves ( d ) LHY ( e ) CCA1 ( f ) PRR family genes. Circles represent PRR1 , triangles represent PRR5 , squares represent PRR7 . Data represented by green lines in c , e , f is from the study by Khan et al . [2] Error bars represent s.d. n =3. * represents significant difference in a t -test, P <0.05. Full size image LER oscillations in continuous light had a hydraulic origin We questioned to what extent oscillations of LER during continuous light are due to plant water movements. Hydraulic conductance and leaf water potential varied synchronously with LER during continuous light in plants previously entrained with large alternations of leaf water potential ( Fig. 2a,b ). Conversely, they were nearly stable in plants entrained with low alternations of leaf water potential ( Fig. 2a,b ). The abundance of ZmPIP aquaporin transcripts in roots varied about synchronously with LER and hydraulic conductance ( Fig. 2c ). Highest oscillation amplitudes of ZmPIP transcript abundance were observed in plants entrained with largest alternations of leaf water potential and transpiration ( Figs 2c and 5 , Supplementary Fig. 6a ), while amplitudes were lower otherwise ( Fig. 2c and Supplementary Fig. 6b ). Transcript abundance showed a minimum at subjective dusk, recovered and reached a maximum at subjective dawn before decreasing again, together with leaf water potential and LER. A peak of transcript abundance was observed 3 h after lights were turned on, regardless of the EP ( Fig. 2c and Supplementary Fig. 6a,b ), probably linked to an intrinsic effect of light or of transpiration on PIP transcript abundance [30] , [31] . All ZmPIP s followed the pattern presented above, except ZmPIP1;4 ( Fig. 5 and Supplementary Fig. 6a,b ). In contrast, no clear oscillation of ZmPIP transcripts abundance was observed in the growing zone of leaves ( Supplementary Fig. 6c ), suggesting that the control of LER oscillations involved PIP expression in roots rather than in leaves. 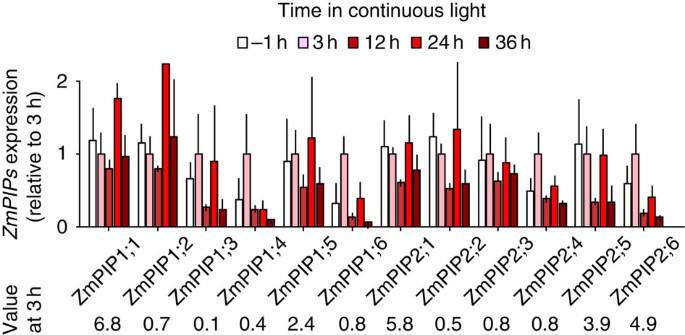Figure 5: The transcript abundance ofZmPIPsaquaporins displayed an endogenous rhythm. IndividualZmPIPs expressions in roots. Error bars represent confidence interval atP<0.05. Other scenarios of EP for roots and transcript abundance in the growing zone of leaves are presented inSupplementary Fig. 6. Figure 5: The transcript abundance of ZmPIPs aquaporins displayed an endogenous rhythm. Individual ZmPIP s expressions in roots. Error bars represent confidence interval at P <0.05. Other scenarios of EP for roots and transcript abundance in the growing zone of leaves are presented in Supplementary Fig. 6 . Full size image In addition to conditions during EP, the amplitude of LER oscillations was affected by genetic or environmental manipulation during continuous light. For given oscillations of transpiration during EP, the amplitude of LER oscillations under continuous light were (i) larger with high than with low evaporative demand ( Fig. 3c , VPD=3 and 0.5 kPa, respectively) and (ii) much larger in hydroponically grown plants at a water potential ( Ψ s ) inducing a water stress ( Fig. 3d , Ψ s =−0.4 and −0.1 MPa, water stress and control conditions, respectively). Plants under-expressing the NCED/VP14 gene (AS) have a lower root hydraulic conductivity, PIP transcript abundance and protein content [19] , and consistently presented larger oscillations of LER than WT during continuous light ( Fig. 3b ). A simulation model was used to test whether changes in plant hydraulic properties may account for the oscillation of LER during continuous light presented in Fig. 1 . It simulates the water transfer from soil to evaporation sites and water potentials in the soil–root interface, xylem, bundle sheaths and mature cells, together with stomatal conductance, leaf growth rate and ABA concentration in the xylem sap [15] . A circadian-driven root hydraulic conductance was superimposed to the light-driven hydraulic conductance already present in the model [15] ( Fig. 6g–i ). Simulated circadian and light-driven root conductances had nearly opposite variations during EP, whereas the circadian-driven oscillation of conductance was the only cause of variation during continuous light, with a simulated amplitude depending on xylem water potential during EP (calibrated on the regression lines in Supplementary Fig. 3a,b ). Overall, the model captured the major patterns of experimental results presented in Fig. 1 ( Fig. 6 ) and on those in ref. 15 ( Supplementary Fig. 10 ). In particular, it captured the contrasting oscillations of LER and of leaf water potential in continuous light depending on the level of evaporative demand during EP and, for a given scenario during EP, the larger amplitudes of LER oscillations with high evaporative demand during continuous light. 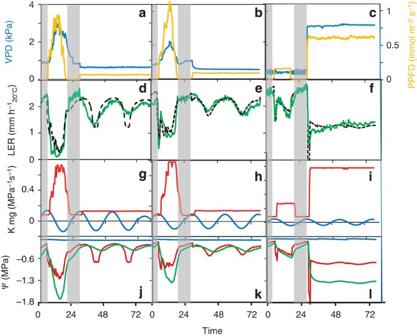Figure 6: A hydraulic model involving oscillations of hydraulic conductance captures experimental patterns of leaf growth and leaf water potential in experiments 11, 12 and 21. (a–c) Photosynthetic photon flux density (PPFD) and air vapour pressure deficit (VPD). (d–f) Leaf elongation rate (LER). (g–i) hydraulic conductance controlled by light (red) or circadian movements (blue). (j–l) Water potentials of the xylem (red) and mature cells (green). Ind–f, green lines represent measured LER, black lines: simulated LER.a,d,g,j: experiment 11.b,e,h,k: experiment 12.c,f,i,l: experiment 21. Figure 6: A hydraulic model involving oscillations of hydraulic conductance captures experimental patterns of leaf growth and leaf water potential in experiments 11, 12 and 21. ( a – c ) Photosynthetic photon flux density (PPFD) and air vapour pressure deficit (VPD). ( d – f ) Leaf elongation rate (LER). ( g – i ) hydraulic conductance controlled by light (red) or circadian movements (blue). ( j – l ) Water potentials of the xylem (red) and mature cells (green). In d – f , green lines represent measured LER, black lines: simulated LER. a , d , g , j : experiment 11. b , e , h , k : experiment 12. c , f , i , l : experiment 21. Full size image No clear alternative mechanism arose from our analyses We have tested whether light signals mediated by phytochromes [32] , [33] , [34] affect rhythmic growth in maize, as they do in A. thaliana [5] . We have used for that the maize mutant elm1 deficient in phytochromes [35] . This mutant presented an oscillating LER ( Supplementary Fig. 7a ) in contrast to the corresponding mutant hy2 of A. thaliana [5] . Other mutants deficient in phytochrome B [36] also presented oscillations of LER in continuous light, similar to those in the null transformants ( Supplementary Fig. 7b–e ). Because these plants presented the etiolating symptoms described in previous studies [35] , [36] , these results question the role of phytochromes in the control of maize rhythmic growth. Both sensitivity of flowering time to photoperiod and rhythmic growth are regulated by the core oscillator of A. thaliana [4] , [5] . In maize, we observed rhythmic growth in a tropical line whose flowering time is photoperiod sensitive, but also in three photoperiod-insensitive temperate lines originating from independent selections for temperate conditions [37] ( Supplementary Fig. 8 ). Hence, temperate lines lost sensitivity to photoperiod for flower induction but not for rhythmic growth. Finally, genes involved in cell-wall relaxation [20] or sugar homoeostasis [38] did not vary consistently with leaf growth during continuous light in our data or in a published transcriptome [2] . Twenty-three putative genes involved in cell-wall relaxation [20] varied significantly, including one expansin and one xyloglucan endotransglucosylase/hydrolase ( Supplementary Fig. 9 and Supplementary Table 2 ), but three genes encoding the expansins best associated with maize leaf growth [39] did not. Eight (out of 917) genes involved in sugar homoeostasis [38] varied in our data, including 1 out of 19 genes involved in starch synthesis and degradation [38] ( Supplementary Table 2 ). Overall, in contrast to core oscillator genes and PIP genes in roots, the oscillations of expression of other genes potentially involved in leaf growth were not straightforward and only PIP transcripts were clearly affected by adverse water conditions during EP. Adaptive advantage of oscillations of hydraulic conductance We have used the simulation model presented above ( Fig. 6 ) to evaluate the interest of the hydraulic control of circadian oscillations of plant hydraulic conductance for plant performance in natural conditions. High oscillation amplitudes had a detrimental effect on simulated growth and photosynthesis over 14 days in all situations mimicking pot experiments presented in Figs 1 and 2 and Supplementary Fig. 10 (effects ranging from −15 to −18% for LER and from −5 to −8% for photosynthesis). This result applied to a large range of evaporative demands, light and soil water status, including scenarios with water stress. The control of oscillation amplitude of root hydraulic conductance may therefore have a role in stress avoidance because it restricts leaf growth in water deficit, thereby decreasing transpiration and saving soil water for later stages of the plant cycle [40] , while it maintains leaf growth at its maximum in favourable conditions by avoiding large oscillations of root hydraulic conductance. However, the decrease in growth and photosynthesis with oscillation amplitude is such that it would be detrimental in most drought scenarios [40] . We therefore suggest that increasing the oscillation amplitude of root hydraulic conductance is probably not a straightforward acclimation process. We have then considered the possibility that the ‘dialogue’ between diurnal changes in plant hydraulic conductance and soil hydraulic conductivity affects root water uptake in soil–root systems including a rhizosphere and a bulk soil [41] . Water continuously flows from the bulk soil to the root system through the rhizosphere, following the gradient of soil water potential [42] , [43] . This flow is slowed down when the rhizosphere dries, consistent with experimental measurements of large differences in water potential over some centimeters, and with models of water transfer [44] , [45] . The decrease in water flow is due to the fact that soil hydraulic conductivity decreases by several orders of magnitude with soil water content, so a dry rhizosphere becomes almost impermeable to water [45] . A temporarily high water uptake can, therefore, have detrimental consequences on 24-h water uptake by considerably and almost irreversibly decreasing the hydraulic conductivity of the rhizosphere [41] , [45] . Decreasing root water uptake during the afternoon (time at which transpiration rate is maximum) has a transitory negative effect on plant water status, but may avoid an excessive dehydration of the rhizosphere that would dramatically decrease its hydraulic conductivity [41] , [45] . Hence, we have questioned if a circadian-driven temporary decrease in root hydraulic conductance during the afternoon can increase the overall 24-h water uptake. This was tested in a system that mimics a field soil in which soil is split into three regions according to the distance from the nearest root (<1 mm, from 1 to 4 cm, and >4 cm from any root, ‘bulk soil’) [46] . Simulations were run in two climatic scenarios ( Fig. 7a,b ), either with unfavourable water conditions involving high evaporative demand and a progressive soil water deficit (Nérac, South France), or with favourable water conditions involving small rainfall and low evaporative demand (Karlsruhe, Germany). Consistent with above paragraphs, low and high oscillations amplitudes of root hydraulic conductance are expected in Karlsruhe and Nérac, respectively, but both amplitudes were simulated in both sites to test their respective interests (red and green traces in Fig. 7 ). 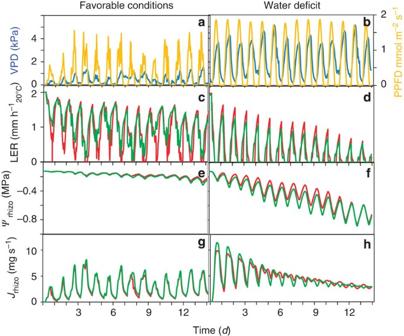Figure 7: Comparative advantages of high or low oscillation amplitudes of root hydraulic conductance in favourable or unfavourable climatic scenarios for water. In each scenario, red and green lines represent simulations with high and low amplitudes of water potential. (a,b) Photosynthetic photon flux density (PPFD) and air vapour pressure deficit (VPD). (c,d) Leaf elongation rate (LER). (e,f) Water potential of the rhizosphere. (g,h) Water flux from the bulk soil to the rhizosphere. Figure 7: Comparative advantages of high or low oscillation amplitudes of root hydraulic conductance in favourable or unfavourable climatic scenarios for water. In each scenario, red and green lines represent simulations with high and low amplitudes of water potential. ( a , b ) Photosynthetic photon flux density (PPFD) and air vapour pressure deficit (VPD). ( c , d ) Leaf elongation rate (LER). ( e , f ) Water potential of the rhizosphere. ( g , h ) Water flux from the bulk soil to the rhizosphere. Full size image Under water deficit, high oscillation amplitudes of hydraulic conductance favoured the simulated water flux from bulk soil to the rhizosphere compared with low amplitudes (+7%, Fig. 7h ). High water flux lasted longer during the day because of the opposition of phases of root hydraulic conductance and soil hydraulic conductivity ( Fig. 6g,h ), resulting in the maintenance of a higher water potential in the rhizosphere ( Fig. 7d , Supplementary Fig. 11 ) and a lower concentration of ABA in the xylem sap ( Supplementary Fig. 12 ). This in turn improved simulated growth and photosynthesis in water deficit ( Fig. 7f and Supplementary Fig. 12 ), with effects of +16 and +11% for LER and photosynthesis, respectively, from days 3 to 14. The same conclusion applied to other multi-compartment soil systems, either with two compartments or with a bi-layer system. In the favourable scenario, high oscillation amplitudes of root hydraulic conductance decreased simulated growth and photosynthesis ( Fig. 7c and Supplementary Fig. 12 ), with negative effects of −17 and −5% for LER and photosynthesis, respectively. In these conditions, high oscillation amplitude did not appreciably affect the flux between bulk soil and rhizosphere ( Fig. 7g ) because soil water potential in the rhizosphere remained at high values ( Fig. 7e , Supplementary Fig. 11 ). Conversely, it affected xylem water potential ( Supplementary Fig. 11 ), leaf growth ( Fig. 7c ) and photosynthesis ( Supplementary Fig. 12 ) during the afternoon, resulting in overall decreases in simulated growth and photosynthesis, as it did in pot experiments. Both experimental data and simulations suggest that oscillations of LER during continuous light were due to rhythmic changes in the plant hydraulic properties, themselves controlled by the amplitude of alternations of xylem water potential during the EP. While circadian oscillations of aquaporin expression have been described in A. thaliana [47] , we show here that they dramatically depend on the level of water stress during EP, and that they have large effects on LER. For a given set of conditions during EP, the amplitude of oscillations under continuous light increased with water tension in the xylem caused by decreased hydraulic conductivity (NCED plants), decreased water potential (experiment with low water potential in hydroponics) or increased water flux through the plant (NCED plants and variations of VPD). The dependence of circadian rythmic growth on hydraulic conditions during EP probably explains the fact that no rythmmic growth has been previously reported in maize and rice [6] , [13] , probably due to the low evaporative demand during EP in these studies, which were performed in standard growth chambers. Simulations of plant behaviours in favourable and unfavourable water scenarios raise the possibility that water stress-dependent circadian oscillations of root hydraulic conductance are one of the mechanisms conferring competitive advantage to plants able to anticipate daily environmental variations and to synchronize growth with them [4] , [8] , [9] . We propose that this mechanism participates in drought tolerance while minimizing the trade-offs usually associated with it [40] , thereby providing an advantage to plants able to anticipate hydraulic variations. High oscillation amplitude, entrained by a period with water deficit, would favour plant water uptake in moderately dry soil. This increases growth and photosynthesis, in spite of an intrinsic negative effect at a given soil water potential of the rhizosphere as observed in pot experiments. Conversely, low oscillation amplitudes entrained by a period with favourable conditions would favour growth and photosynthesis in plants grown in a wet soil. We are aware that this conclusion originates from a model, but these mechanisms would be nearly impossible to detect via an experimental approach. They could be confirmed experimentally with plants whose circadian oscillations of hydraulic conductance are dramatically altered or abolished without deleterious effects on other plant functions, which do not currently exist. Plant materials and growth conditions Experiments were performed with line B73 (temperate, dent), compared with lines CML69 (tropical), F2 (temperate, early French flint) and W22 (temperate, dent). It was also compared with a near isogenic line introgressed in chromosome 5 with a 120 Mbp genomic region originating from a tropical line that presents lower day–night alternations of LER than B73 (ref. 24 ). One NCED antisense maize line [19] was compared with its null transformant (A188 background). The phytochrome-deficient maize mutant elongated mesocotyl 1 ( elm1 ; ref. 35 ) and the mutants phyB1 , phyB2 and the double mutant phB1phyB2 (ref. 36 ) were compared with their null transformant (W22). These plants were severely etiolated in our experiments, with symptoms similar to those described in a previous study [36] . Twenty-two experiments, including 21 experiments with line B73, were carried out with contrasting conditions during the EP (≥96 h) and during the period with continuous light (48 h), as presented in Supplementary Table 1 . Plants were grown and measured during the EP in the Phenodyn platform ( http://bioweb.supagro.inra.fr/phenodyn/ [48] as described previously [15] . Air temperature, temperature of the meristematic region, photosynthetic photon flux density (PPFD) and leaf-to-air vapour pressure difference (VPD la ) were recorded every 15 min (ref. 15 ). The EP occurred either in the green house or in the growth chamber depending on experiments ( Supplementary Table 1 ). In the latter case, plants were transferred from the green house to the growth chamber during the night, using green light, 8 h before the onset of light in the growth chamber. Night temperature was 20 °C (same as in green house) and VPD was 0.8 kPa. The light onset in the growth chamber was matched with sunrise in the green house, with values of PPFD reported in Supplementary Table S1 . The temperature was increased to 28 °C when lights were turned on and was kept constant during the continuous light period for all experiments. VPDs are reported in Supplementary Table S1 for all experiments. Experiments 1–12 (green house) and 19–22 (growth chamber) were carried out with soil 1, containing a 40:60 (v/v) mixture of filtered loamy soil (particle diameter ranging from 0.1 to 4 mm) and organic compost. Experiment 13–16 were carried out with soil 2 (30% clay, 70% peat), which causes lower day/night oscillation amplitudes of LER than soil 1, because of a higher hydraulic conductivity [49] . In both cases, soil water content was determined by automatically weighing columns every 15 min. Soil water potential was estimated according to water content and water release curves of either soil [15] . The soil was maintained at water potentials ranging from 0 to −0.1 MPa by daily watering. In experiments 7 and 18, maize seedlings were grown in hydroponics with a nutrient solution presented earlier [15] . Maize seedlings were placed in tubes with mineral fibres and transferred to the green house with their roots bathing in a continuously aerated solution [15] . The hydroponic solution was renewed every third day and the pH was controlled every day. A mannitol treatment was imposed by replacing the standard nutrient solution by a nutrient solution containing 28.6 g l −1 mannitol (mannitol; Sigma-Aldrich, St Louis, MO, USA) corresponding to a water potential of −0.4 MPa checked with a vapour pressure osmometer (Vapro 5520; Wescor Inc., Logan, UT, USA). Mannitol treatment was applied during the dark period 12 h before the light was switched on. In this experiment, the nutrient solution was renewed every 24 h. Other environmental data were measured and stored as above. LER was measured as presented earlier [15] when the tip of the sixth leaf appeared above the whorl and lasted until the appearance of leaf 8. During both EP and continuous light, the amplitude of oscillations was calculated as ((LER max —LER min )/LER max ), where LER max and LER min are the maximum and minimum values of LER, respectively. In continuous light, subjective dusks and dawn were defined as the times at which LER were minimum and maximum, respectively ( Fig. 1d ). In this calculation, values of LER were averaged over 3 h around minimum or maximum, and over two consecutive subjective dusks during EP. Transpiration rate was estimated every 15 min from the change in pot weight [15] . Leaf water potential was measured [15] at pre-dawn and every 12 h in experiments 4, 9 and 21. Gas exchanges were measured every minute on the fully developed fifth leaf of one plant during 48 h with a gas analyzer (LI-6400, LICOR, Lincoln, NE, USA), and every hour in the same leaf of 10 plants with a diffusion porometer (AP4; Delta-T Devices) calibrated every 30 min. Only measurements performed with high and medium evaporative demands provided consistent data and are presented here (experiment 4). Quantitative RT–PCR and transcriptome analysis Six-cm-long elongating tissues of leaves 7, 8 and 9, and the 5 cm behind root tips were sampled 1 h before light and every 12 h after the light was turned on (peaks of LER oscillations) in experiments 3, 20 and 21, with three (experiment 3) or four (experiments 20 and 21) biological replicates. RNA extraction, complementary DNA synthesis and real-time PCR were performed as previously described [50] . Data were analyzed by the 2 −ΔΔCt method [51] and normalized using three reference genes, ACT1 (accession number gi: 450292), EF1-α (gi: 2282583) and polyubiquitin (gi: 248338). The oligonucleotide microarray Maïs 45K BGA (Roche NimbleGen Inc., Madison, WI, USA) was processed and analyzed as in ref. 15 . Three samples of the leaf growing zone were collected 1 h before the light was turned on, 12 and 24 h after it in experiment 4. Total RNA, RNA integrity, complementary DNA synthesis, purification and labelling, overnight hybridization (16 h at 42 °C) and laser acquisitions were performed as earlier [15] . Intensities were extracted, filtered and normalized with the NimbleScan software. Raw hybridization intensities were normalized across all arrays with Robust Multichip Average Express (RMA) in which the quantile normalization method was employed [52] . Data were imported into R (R Core Team, 2013, http://www.R-project.org ). Change with time in transcript abundance corresponding to a given probe was considered as significant if (i) the P -value was <0.05 in a t -test and (ii) it differed by a factor >1.5 between times of sampling. Values shown in Fig. 4 and Supplementary Fig. S9 are log 2 ( t 0 / t n ), where t 0 and t n are the values at dawn and at time n . Functional annotation was enriched with homologous genes of other species identified by BLASTp against plant protein sequences from Uniprot ( http://www.uniprot.org/ ) and Rice Protein sequences (MSU Rice Genome Annotation Project Release 6.0). The classes of genes presented in Supplementary Fig. 3 were prepared following the ontologies of MapMan ( http://gabi.rzpd.de/projects/MapMan ) for maize Zm_B73_5b_FGS_cds_2012 ( http://mapman.gabipd.org/web/guest/mapmanstore ). Transcript analyses of plants grown under low evaporative demand (entrainment and continuous light) were obtained from a published study [2] . The day VPD calculated from author’s data was 1 kPa, with a photoperiod of 12 h light and 12 h dark. The data set containing the normalized expression values of each probe and the functional annotation of maize transcripts in the microarray was obtained from ( http://www.biomedcentral.com/1471-2229/10/126 ). Model of water transfer The model is derived from that of Tardieu and Davies [53] run at a time step of 1 min ( Supplementary Fig. 13 ). Water flows from soil to air via plant compartments, following gradients of water potential from the rhizosphere ( Ψ rhiz ) to roots ( Ψ r ), xylem ( Ψ xyl ) and bundle sheaths ( Ψ bundle ). The water flux can be diverted to a capacitance representing mature leaf tissues ( Ψ leaf ). We have argued that Ψ leaf is the water potential measured with a pressure chamber [15] . Ψ xyl stands for the water potential in the leaf xylem near the leaf insertion point, close to the leaf elongating zone. Root water potential ( Ψ r ) stands for the water potential at the outer root surface. The water potential in the rhizosphere ( Ψ rhiz ) is an equivalent of that proposed [54] to represent the water potential of the soil surrounding roots during the night, close to pre-dawn water potential. We have mimicked the water transfer simulated by a three-dimensional model of water transfer [42] ( Supplementary Fig. 14 ) by considering three interlocked cylinders. The first one, in which all the soil is at less <1 mm from any root is represented by a cylinder of 0.1 m radius and 0.5 m depth, in which the distance between roots is calculated from root length and resistance to water transfer is calculated using equation 3. The second cylinder represents the soil localized at <4 cm from the nearest root, with a diameter of 0.14 m and a depth of 0.54 m ( Supplementary Fig. 14 ). The third cylinder (0.26 m diameter, 1.6 m depth) represents the ‘bulk soil’ available to one plant. The latter is the product of the soil area occupied by one plant, that is, the reciprocal of plant density (7.6 plant per m 2 ) by soil depth. These respective volumes were consistent with those measured in a maize field from maps of root impacts on six horizontal planes [55] ( Supplementary Fig. 14 ). In each compartment, Ψ soil is related to soil water content (W) and soil hydraulic conductivity is related to Ψ soil by using the Van Genuchten equations [56] Where n , α, ks and p are coefficients that characterize a given soil texture [56] , with values 1.21, 3.21, 0.1 and 0.5, respectively. Potentials are expressed in MPa. The resistance R sp (MPa s mg −1 ) between the rhizospere and soil–root interface was calculated as in ref. 57 where d and r are the mean distance between neighbouring roots and root radius, respectively, in the rhizosphere volume. k ( Ψ soil ) is the soil hydraulic conductivity in the same compartment. The fluxes J soil1 and J soil2 between compartments were calculated as Where r col and prof col are the radius and depths of the first column (see Supplementary Fig. 14 ). The conductance to water transfer from the soil–root interface to the xylem (Gr, mg MPa −1 s −1 per plant) depends linearly on the amount of light received by the plant (PPFD), with a maximum value and a delay (set by default at 90 min). This delay accounts for the transient decrease in leaf growth observed when light is turned on in growth chamber experiments [58] . G r is the sum of G r_lum and an oscillating conductance ( G r_circad) Where time photo is the time in the photoperiod. Ψ xyl min and Ψ xyl max are the minimum and maximum Ψ xyl during the considered EP. A resistance R xl (MPa s mg −1 ) connects Ψ xyl to the water potential of bundle sheaths ( Ψ bundle ). Ψ bundle is the water potential assumed to affect stomatal conductance in equation 8. Mature tissues are represented by a compartment that has a capacitance and is related to Ψ bundle with a conductance G c (mg MPa −1 s −1 ). The capacitance and G c were fitted on the results of a rehydration experiment [15] . The flux J xc (mg per plant per s) between mature tissues and bundle sheaths was calculated following the gradient of water potential between both compartments and the conductance G c . The latter is considered to depend on PPFD in the same way as G r . We therefore solved the differential equation for calculating the cell water potential Ψ cel and J xc . where V sat (mm 3 ) is the leaf volume at saturation and V res is the residual water volume −0.3 MPa, α and n are the parameters of a Van Genuchten equation fitted on the pressure volume curve (values: 0.075 and 1.5, respectively). J xc was calculated as the difference in V cell between two different times for the optimization process of resolution of the differential equation. At each time i , the flux through roots and xylem is the sum of the transpiration flux J and of J xc . The model calculates stomatal conductance, the concentration of ABA in the xylem sap [ABA] xyl , water flux, root and the water potentials in transpiration sites from soil water potential, light intensity and air VPD. Stomatal conductance is calculated as in ref. 53 . where g smin is the minimum stomatal conductance resulting from cuticular conductance and conductance through closed stomata. α , β and δ are the parameters for maize [53] (values: 0.182, −0.003 and −1, respectively). The transpiration flux J is calculated with the Penman Monteith equation but taking into account plant leaf area to express transpiration per plant ( Supplementary Fig. 13 ). [ABA] xyl is calculated as in ref. 53 . The model first solves every minute the five equations with five unknowns, namely the Penman Monteith equation ( Supplementary Fig. 13 ), equations 10 and 11 and the equations relating the water flux to the difference in potential between Ψ bundle and Ψ r divided by the resistance R p and that relating the water flux to the difference in potential between Ψ rhizo and Ψ r ( Supplementary Fig. 13 ). It then solves equations 8 and 9. LER is calculated as a maximum rate, genotype dependent, which is affected by ln [ABA] xyl as in ref. 59 , with a linear effect (a_r_aba) and by Ψ xyl in a linear manner (parameters a_ler and c_ler), as in ref. 60 (values 3.5 and 0.8, respectively). It is noteworthy that [ABA] xyl has a very small effect compared with Ψ xyl . Photosynthesis can be calculated from stomatal conductance [61] . The model is implemented in the R language. Simulations were run with this model using time series collected in experiments conducted in Nérac and Karlsruhe in July 2012. Environmental data were collected daily in both sites every hour, namely air temperature, air relative humidity, incident light and rainfall. Experiments with B73 provided maize yields of 12.1 T ha −1 and 5.1 T ha −1 in Karlsruhe and Nérac, respectively. Two amplitudes of Ψ xyl were used, namely 0.2 and 0.8 MPa in each site. The plant density in the model was similar to those in the corresponding experiments (7.6 m −2 ) and soil depth was 1.6 m. Leaf area per plant used in simulations was 0.8 m 2 , a realistic value for maize plants at flowering time. It did not change with time in simulations because leaf growth has already stopped at that time of the plant cycle. How to cite this article : Caldeira, C. F. et al . Circadian rhythms of hydraulic conductance and growth are enhanced by drought and improve plant performance. Nat. Commun. 5:5365 doi: 10.1038/ncomms6365 (2014). Accession codes: Microarray data has been deposited in the NCBI GEO database with accession code GSE55524 .